Origami-like unfolding of hydro-actuated ice plant seed capsules Actuated plant materials are a source of inspiration for the design of adaptive materials and structures that are responsive to specific external stimuli. Hydro-responsive, metabolism-independent plant movements are particularly fascinating, because the extracted concepts are more amenable to transfer into engineering than those dependent on cellular activity. Here we investigate the structural and compositional basis of a sophisticated plant movement mechanism—the hydration-dependent unfolding of ice plant seed capsules. This reversible origami-like folding pattern proceeds via a cooperative flexing-and-packing mechanism actuated by a swellable cellulose layer filling specialized plant cells. Swelling is translated into a bidirectional organ movement through simple geometric constraints embedded in the hierarchical architecture of the ice plant valves. Extracted principles from this reliable and reversible actuated movement have relevance to the emerging field of 'programmable matter' with applications as far-reaching as the design of satellites and artificial muscles. Water is the medium of life; nevertheless, certain organisms have evolved impressive adaptations not only to survive, but also to prosper in environments with scarce water resources. The Aizoaceae , with many species commonly known as ice plants, have demonstrated exemplary evolutionary radiation in arid and semi-arid habitats [1] . Central to their success is a distinctive seed dispersal mechanism in which protective valves on their seed capsules mechanically open only when sufficiently hydrated with liquid water ( Fig. 1a,b,c ), thus increasing the likelihood that seeds will be dispersed under conditions favourable to germination [2] . This complex and directed movement is especially fascinating because the seed capsules at this point are non-living. This differs from traditional osmotically driven plant movements, exemplified by Venus fly traps [3] , [4] or plant stomata [5] , and resembles more the passive movements of wheat awns [6] or pine cones [7] . In these latter two cases, a bending movement during drying and rewetting is achieved by a bilayered structure in which opposing tissues possess different cellulose fibril orientations in their cell walls. This results in varying amounts of axial deformation of the cell wall in each tissue type on shrinking or swelling of the matrix polymers, as the composite deforms not along but perpendicular to the cellulose fibril orientation. However, using this kind of structural organization, only relatively simple bending movements can be achieved. The unfolding of the ice plants is also hydration dependent; but, as will be demonstrated, the sophisticated hierarchical structuring of the seed capsules allows for a more complex origami-like unfolding movement that incorporates an effective flexing-and-packing mechanism. 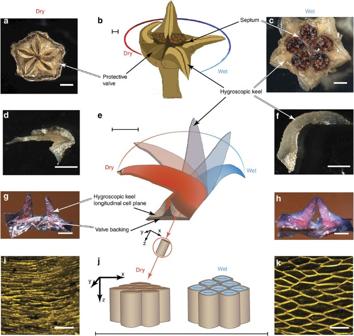Figure 1: Ice plant seed capsule hierarchical morphology. Light and confocal microscopy images depict the morphology of the ice plant capsule and the hygroscopic keel tissue at different hierarchical levels (a–k). For each hierarchical level, an illustrated schematic provides a simplified representation of structures and the progressive movements that occur during water-dependent actuation. Cell longitudinal images (g,h) were stained with FCA to provide contrast. Contrast in confocal images (i,k) originates from lignin autofluorescence. Scale bars are defined as follows:aandc=2 mm;b,eandj≈1 mm;dandf=1 mm;gandh=0.5 mm;iandk=0.1 mm. Figure 1: Ice plant seed capsule hierarchical morphology. Light and confocal microscopy images depict the morphology of the ice plant capsule and the hygroscopic keel tissue at different hierarchical levels ( a – k ). For each hierarchical level, an illustrated schematic provides a simplified representation of structures and the progressive movements that occur during water-dependent actuation. Cell longitudinal images ( g , h ) were stained with FCA to provide contrast. Contrast in confocal images ( i , k ) originates from lignin autofluorescence. Scale bars are defined as follows: a and c =2 mm; b , e and j ≈1 mm; d and f =1 mm; g and h =0.5 mm; i and k =0.1 mm. Full size image Here we utilize a multidisciplinary approach at various hierarchical levels to investigate the unfolding mechanism of the desert ice plant seed capsule from the species Delosperma nakurense (Engl.) Herre. Our results indicate that the actuation of the seed capsule valve is mediated by a swellable cellulose layer in specialized cells and translated into a sophisticated bidirectional unfolding movement by the geometry of the cells and their hierarchical arrangement. Morphological characterization of seed capsules Figure 1 summarizes the hierarchical structure of the seed capsule from D. nakurense in the dry and hydrated state and provides a schematic representation of the three-dimensional structure at each level. The axes in the schematics are defined relative to the position and orientation of the keel and its cells. In the dry state, five protective valves cover the seed compartments, preventing premature dispersion of seeds ( Fig. 1a ). When hydrated with liquid water, each valve unfolds outwards and backwards over an angle of ∼ 150° within minutes ( Fig. 1a–c ; Supplementary Movie 1 ). Seed compartments are partitioned by five septa, which lie beneath the centre of each valve in the closed dry state. The schematic in Figure 1b is a 3D illustration of the whole capsule in which each valve is depicted at a different stage of opening, to provide a more intuitive representation of the subsequent steps involved in the unfolding process. The hygroscopic keel, a prominent tissue attached along the centre of the inner valve surface can clearly be seen in Figure 1c and was previously suggested to actuate this water-dependent movement [8] , [9] . The reversible water-actuated flexing movement of the keel can still be observed even when it is dissected from the backing ( Fig. 1d–f ; Supplementary Movies 2 and 3 ). The schematic in Figure 1e further illustrates the progression of this movement, which occurs over a time scale of a couple of minutes. The keel consists of two separated halves with single cells of different lengths running from the top to the bottom of the keel (the longitudinal axis of the cell is assigned as the Z-direction) ( Fig. 1e,g,h ). The two halves of the keel are separated in the dry state, but come into contact by swelling when hydrated, creating a bridge-like structure with an empty space between the upper portion of the keel and valve backing ( Fig. 1g,h ). Additionally, changes in the hydration state appear to result in a curvature of the valve backing in the dry state and straightening in the wet state ( Supplementary Movie 4 ). Transverse sections of keels reveal a lattice structure with hexagonal/elliptical shaped cells in the wet state. When dried, the elliptical shaped cells are collapsed preferentially in the shorter axis of the transverse cell cross-section, which we assign as the Y-direction ( Fig. 1i–k ). Consequently, the longer axis of the transverse cell cross-section is assigned the X-direction. The orientation of the cells within the larger keel structure, as well as the hydration-dependent changes in shape, is depicted in the schematic in Figure 1 j. The stepwise changes in the keel during drying were examined in more detail using image correlation to track the progressive movements ( Fig. 2 ). 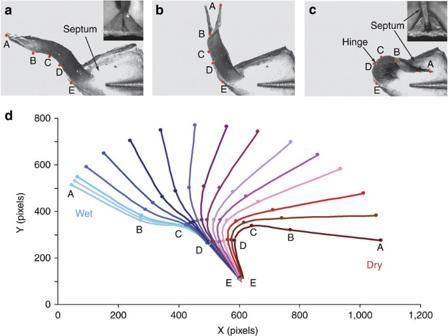Figure 2: Detailed analysis of keel movement. Image correlation was used to track the movement of a dissected keel during drying. A keel attached to the septum with the backing dissected away can be seen in the wet state (a), an intermediate state (b), and the dry state (c). The red spots labelled A–E were followed in consecutive frames to observe the relative movements of the keel. Insets (a,c) show the tight packing of the keel around the septum in the dry state. (d) plot of relative movements of points A–E during drying. From the plot in Figure 2d, it is apparent that the tip of the keel (point A) is translated about the base (point E) through a large angle. Additionally, there is a point of maximum bending in the keel in the dry state, located between points C and D in Figure 2c , that we define as the 'hinge' of the flexing movement. It is also clear from the insets in Figure 2a,c (cut made through the keel between points D and E) that the gap between the two keel halves in the dry state allows them to fit tightly around the septum as they close, without being obstructed. Because the valves are closed during development, the gap between the keels in the dry state represents the initial conformation and seems to be a prerequisite for a tight packing of the valve. Figure 2: Detailed analysis of keel movement. Image correlation was used to track the movement of a dissected keel during drying. A keel attached to the septum with the backing dissected away can be seen in the wet state ( a ), an intermediate state ( b ), and the dry state ( c ). The red spots labelled A–E were followed in consecutive frames to observe the relative movements of the keel. Insets ( a , c ) show the tight packing of the keel around the septum in the dry state. ( d ) plot of relative movements of points A–E during drying. Full size image Morphology and composition of hygroscopic keel cells The large and directed change in the Y-direction of keel cells upon hydration indicates that the flexing movement of the keel originates at the cell and cell wall level. In fact, cells show a highly anisotropic deformation with a fourfold increase in length along the Y-direction (short cross-sectional cell axis) whereas the X-direction (long cross-sectional cell axis) length shows only minor changes ( Table 1 ). This is accompanied by a nearly fourfold enlargement of the cross-sectional area and a modest increase in the perimeter ( Table 1 ). Additionally, it was observed that the cell length in the Y-direction of the expanded wet state was 20% lower in keel cells attached to the backing ( Fig. 1e,g,h ) than in those near the ridge of the keel ( T -test P <0.005). This asymmetrical deformation facilitates the bending of the keel during cell swelling. Table 1 Transverse cell shape changes during wetting and drying cycles. Full size table Cell wall organization and composition were investigated by staining with a fuchsin-chrysoidin-astra blue mixture (FCA), which revealed lignified cell walls (red staining) and a non-lignified cellulose structure filling the lumina (bright blue staining) ( Fig. 3a ). Further characterization with confocal Raman spectroscopy ( Fig. 3b–e ) corroborated these observations. The main Raman peaks for cellulose appear in both the cell wall and the inner layer, whereas the lignin peak appears only in the cell wall and between cells ( Fig. 3b–d ). Whereas the inner layer, which we will hereby refer to as the cellulosic inner layer (CIL), may contain additional biomacromolecules such as pectin or hemicelluloses in smaller amounts [10] , [11] , it is most important for this study that the CIL can apparently absorb large amounts of water ( Fig. 3e ). Additionally, the CIL appears to be organized as thin lamellae running parallel to the X-direction ( Fig. 3c ). Consecutive laser scanning confocal microscopy images of drying keel cells in which the cell wall and CIL are differentially stained reveal that, during cell collapse, the CIL retracts towards and remains attached to the surrounding cell wall ( Fig. 3f–h ; Supplementary Movie 5 ), suggesting the CIL may have an active role in the reversible actuated cell deformation. 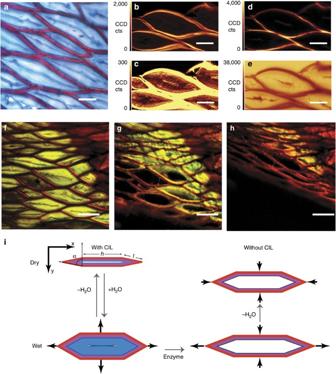Figure 3: Biomolecular composition of hygroscopic keel cells. (a) FCA staining reveals a lignified thin cell wall (red) and a CIL in the cell lumen (blue). (b–e) Confocal Raman spectroscopic images of keel cells integrated for cellulose (bandc, 1,067–1,143 cm−1) at two different intensity levels, lignin (d, 1,546–1,643 cm−1), and water (e, 2,223–2,725 cm−1). (f–h) Consecutive confocal microscopy images of safranine-stained keel cells during drying, coloured to differentiate between the cell wall (red) and CIL (green-yellow). (i) Schematic of changes in keel cell cross-sectional shape following treatments. Relative cell shapes are represented as idealized hexagons with the appropriate ratios of X to Y lengths. Thick black arrows represent the direction of change in the X and Y lengths of the cell following the respective treatment. Scale bars are defined as follows:a=25 μm;b–d=20 μm;f–h=50 μm. CCD, cts, Figure 3: Biomolecular composition of hygroscopic keel cells. ( a ) FCA staining reveals a lignified thin cell wall (red) and a CIL in the cell lumen (blue). ( b – e ) Confocal Raman spectroscopic images of keel cells integrated for cellulose ( b and c , 1,067–1,143 cm −1 ) at two different intensity levels, lignin ( d , 1,546–1,643 cm −1 ), and water ( e , 2,223–2,725 cm −1 ). ( f – h ) Consecutive confocal microscopy images of safranine-stained keel cells during drying, coloured to differentiate between the cell wall (red) and CIL (green-yellow). ( i ) Schematic of changes in keel cell cross-sectional shape following treatments. Relative cell shapes are represented as idealized hexagons with the appropriate ratios of X to Y lengths. Thick black arrows represent the direction of change in the X and Y lengths of the cell following the respective treatment. Scale bars are defined as follows: a =25 μm; b – d =20 μm; f – h =50 μm. CCD, cts, Full size image Mechanics of hygroscopic keel cell swelling Following enzymatic removal of the CIL, cells largely lose the ability to close during drying ( Fig. 3i and Table 2 ). In addition, removal of the CIL in the wet state results in a cell-shape relaxation in which the Y-length decreases and the X-length increases ( Fig. 3i and Table 2 ). These observations suggest that the CIL has a role in both closing and opening of the cells. Specifically, the hydrated CIL may generate outward stresses on the cell wall through an internal pressure during swelling, thus facilitating the cell opening. For this particular mechanism to function, it would be necessary for the cells to deform more easily in the Y- than X-direction. In fact, calculations of elastic deformability based purely on geometrical considerations support this assumption. If we consider keel cells as an ideal cellular solid with a hexagonal shape as depicted in Figure 3i , the ratio of stiffness in the X- and Y-direction can be calculated according to equation (1) derived from Gibson & Ashby [12] . Table 2 Relative changes in cell dimensions due to hydration changes and enzymatic removal of CIL. Full size table Based on the anatomical cell parameters measured in the dry keel ( Fig. 3i and Table 1 ) and under the simplifying assumption of isotropic cell wall material, the keel tissue would be ∼ 5,500 times stiffer in the X-direction than in the Y-direction. When the cells are in the wet open state, this factor decreases to a value of only ∼ 30. This mechanical and geometrical anisotropy is consistent with a CIL-driven mechanism of keel cell opening. Additionally, the apparent lamellar structure of the CIL may lead to an anisotropic swelling which would further facilitate the deformation in the Y-direction; however, based on our calculations, this is not necessarily required. Characterization of valve curvature In addition to the flexing deformation of the valve described above, we also observe a change in the curvature of the valve backing in the XZ-plane, which may be important for the opening mechanism ( Fig. 4 ). In the dry state, the backing shows a concave-curved morphology, which appears to be related to the gap formed between the two keel halves and thus important for tight valve packing ( Figs 2c and 4 ). The curvature exists from the tip of the valve down to the hinge, with a graded reduction in the degree of curvature as one approaches the hinge. 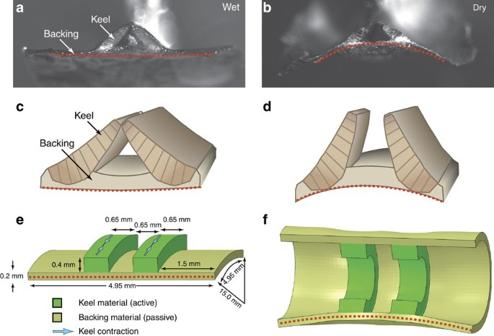Figure 4: Ice plant valve curvatures. aandbshow the change in the curvature of the valve backing in the XZ-plane in the wet and dry state, respectively, which is represented in schematic form incandd. A finite element model of contractile elements (green) on top of a shell (yellow) demonstrates that contraction of these elements (keels) in the y-direction initiates a curving of the shell (backing) in the XZ-plane (eandf). Scale bars are defined as follows:a=25 μm;b–d=20 μm;f–h=50 μm. Figure 4a,b depicts the curvature in the wet and dry state of the keel backing at the hinge (cut between points C and D as defined in Fig. 2c ). On wetting, the valve backing straightens and the tips of the keel halves move towards each other ( Fig. 4a–d; Supplementary Movie 4 ). When keels have been dissected away from the backing, this change in curvature of the valve is not observed ( Supplementary Movie 6 ), suggesting that the large deformation of the keel in the Y-direction may not only actuate the flexing movement, but may also additionally influence the valve curvature. This effect can be simulated by simple finite element modelling of contractile elements (keels) on top of a shell (backing) ( Fig. 4e,f ). Contraction of the model 'keels' in the Y-direction results in the development of elastic stresses in the shell which are released via a curvature of the shell in the XZ-plane in the expected direction. The magnitude of the curvature varies with shape, thickness and elastic properties of the backing and the keel. Comparable deformation mechanisms have been identified in other shell-like materials such as leaves where stress gradients arising from differences in growth rates within the leaf plane can be relieved by out-of-plane bending [13] , [14] . Figure 4: Ice plant valve curvatures. a and b show the change in the curvature of the valve backing in the XZ-plane in the wet and dry state, respectively, which is represented in schematic form in c and d . A finite element model of contractile elements (green) on top of a shell (yellow) demonstrates that contraction of these elements (keels) in the y-direction initiates a curving of the shell (backing) in the XZ-plane ( e and f ). Scale bars are defined as follows: a =25 μm; b – d =20 μm; f – h =50 μm. Full size image The adaptive behaviour of ice plants ( Aizoaceae ) has been shaped by life in arid and semi-arid environments. Due to the scarcity of water, specific adaptations by the organisms are required that ensure survival and reproduction. A distinct feature of the Aizoaceae is the water-actuated opening of seed capsules for seed dispersal. We have observed that the actuated folding and unfolding of the protective valves in ice plant seed capsules consists of two discrete but coordinated movements, which we assign as flexing and packing, respectively. Morphological and compositional characterization of the hygroscopic keel revealed the presence of a layer of primarily cellulose (CIL) within the ellipsoid cells, which is capable of absorbing large amounts of water. A similar swellable cellulosic layer termed the 'gelatinous layer' has previously been identified as the active element of stress generation in tension wood fibres of hardwood trees [15] , [16] , [17] , [18] , contractile roots [19] , [20] and tendrils [21] . It has been recently proposed to induce plant organ movement by exerting an inner pressure on the surrounding cell wall [22] . The keels of ice plant seed capsules apparently utilize a related principle; however, in this case, the structural optimization is not mediating longitudinal contraction of cells, but, instead, establishing a specific anisotropy in the transverse deformability of the cells. This specific deformation at the cell level is translated into the flexing movement of the keel, which requires a large deformation in the Y-direction (see Fig. 1 ). The second movement contributing to the actuated unfolding mechanism in ice plant seed capsules is the hydration-dependent change in curvature observed in the valve backing. There seems to be a clear link between the curvature of the backing and the gap formed between the two keel halves. In the initial state of the dried capsule before it is opened by hydration, the five septa dividing the seed compartments fit tightly in the gap between the keel halves for each of the five valves ( Fig. 2c ). This implies that the curved backing and the proper packing are closely interrelated in the dry state. However, the curvature of the backing may hinder the unfolding of the valve during wetting. This geometrical constraint is demonstrated through a simple paper-folding experiment ( Fig. 5a–d ; Supplementary Movie 7 ). Curving the top half of a folded sheet of paper stabilizes the 'closed' structure, while straightening releases the folded structure. The efficacy of this mechanism depends on the presence of curvature at the hinge. Transferring this observation to the ice plant capsule implies that a swellable tissue could more easily move the top half about the hinge in an uncurved state because the required force is reduced, analogous to a conceptualized mechanism of the keel as a flexing muscle ( Fig. 5e ). Therefore, we propose that to unfold a valve for seed dispersal, the backing needs to switch from a curved to a plane status. The finite element model ( Fig. 4e,f ) and the paper model ( Fig. 5a–d ) differ in whether or not they allow for stretching deformation of the backing materials, and therefore represent two extreme cases of how the curving deformation may proceed. It is likely that the actual capsule behaviour lies somewhere between these extremes; however, both models provide important reference points for assessing this behaviour. 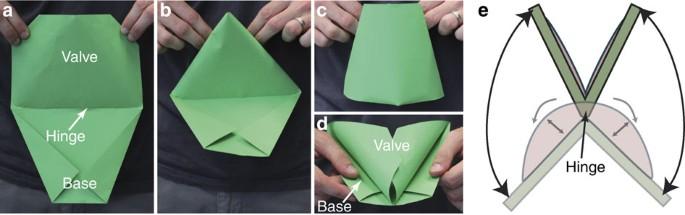Figure 5: Conceptualized mechanism of ice plant valve curvature. (a–d) 'Action' Origami demonstration of the curvature mechanism. When the top half of the folded paper representing the valve is straight (a), it is free to move about the fold (hinge). If the top half is curved by bringing the corners together, the bottom half moves about the hinge towards the top half (b) until both halves are brought together (c). (d) shows the same fold as (c) from another perspective. It was not possible to move the paper about the hinge until the top half was again uncurved. (e) Schematic demonstrating reversible movements of the unlocked bendable substrate actuated by the expansion of a swellable layer. Figure 5: Conceptualized mechanism of ice plant valve curvature. ( a – d ) 'Action' Origami demonstration of the curvature mechanism. When the top half of the folded paper representing the valve is straight ( a ), it is free to move about the fold (hinge). If the top half is curved by bringing the corners together, the bottom half moves about the hinge towards the top half ( b ) until both halves are brought together ( c ). ( d ) shows the same fold as ( c ) from another perspective. It was not possible to move the paper about the hinge until the top half was again uncurved. ( e ) Schematic demonstrating reversible movements of the unlocked bendable substrate actuated by the expansion of a swellable layer. Full size image Seed capsules of ice plants exhibit a complex hydroactive movement, which is mediated by the hygroscopic keel and achieved via a sophisticated interplay between the cell walls and the CIL generating a carefully choreographed unfolding/folding of the whole seed capsule. Two cooperative bidirectional movements have been identified both of which are dependent on the large anisotropic deformation of the keel cells; a flexing of the valve during folding and unfolding, and an out-of-plane curving of the valve backing which facilitates tight packing in the closed state and additionally, may reduce the force for unfolding in the wet, uncurved state. The highly synergistic interplay of both mechanisms under natural conditions becomes obvious when drying is accelerated by applying a vacuum. Under these artificial conditions, open capsules do not close, but get stuck open in the dry state after partially closing. Presumably, a concerted drying sequence of the highly hygroscopic CIL and the less hygroscopic lignified cell walls is crucial to avoid a temporal mismatch of the bidirectional movements. Whereas we can only speculate about the evolutionary function of the water-actuated change in valve curvature, the observed behaviour can provide inspiration for the packing and locking design of novel actuated structures. The cooperative reversible flexing-and-packing of the ice plant capsule resembles self-organized 'action' Origami (for example, the Miura-ori fold that has inspired folding patterns for satellites) [23] , [24] and may assist recent efforts by researchers to create programmable matter which can achieve a specific folded conformation following a stimulus [25] , [26] . Sample preparation Ripe capsules were collected from D. nakurense plants grown at the Botanical Garden of the Technische Universität Dresden, accession nr. 009255-21, and kept dry for storage. Keels were carefully dissected away from the valve backing in the wet state with tweezers and scalpel. For some experiments, pieces of keel tissue were embedded in polyethylene glycol (MW=2,000) and sections ranging in thickness from 10–30 μm were cut with a Leica RM2255 rotation microtome. Sections were washed in distilled water to dissolve and remove the PEG and were used for light microscopy, confocal microscopy, and Raman spectroscopy. Further staining with a solution of FCA was used for contrast and compositional analysis. Additionally, staining with 0.1% aqueous safranine was used for confocal microscopy samples [27] . In both cases, samples were immersed in the staining solution for 5–10 min and then washed three times in distilled water. Cell dimension measurements To quantify changes in the cell shape during wetting and drying cycles, it was necessary to use light microscopy for wet measurements and scanning electron microscopy for dry measurements. Both wet and dry measurements were made from the same region of a single piece of keel. Measurements were made using ImageJ v1.43 l and a computer drawing tablet to determine the length of cells along the X- and Y-directions, as well as their perimeter, and area. Raman spectroscopy Thin sections of keel tissue were fixed under a glass coverslide in distilled water or D 2 O. Raman spectra were collected with a confocal Raman microscope (alpha300; WITec) equipped with a piezoelectric scan stage (P-500, Physik Instrumente) and a Nikon objective (100x oil immersed, NA=1.25) [28] . A laser of λ=532 nm was focused onto the sample and Raman scattering was detected with a CCD camera (DV401-BV; Andor) behind a spectrometer (UHTS 300; WITec) with a spectral resolution of 3 cm −1 . Samples were mapped in 0.33 μm steps using an integration time of 0.5 s. Data were analysed and images were produced using ScanCtrlSpectroscopyPlus software (WITec). Confocal microscopy Laser scanning confocal microscopic imaging was performed with Zeiss LSM 510 scanning system (Zeiss MicroImaging GmbH) equipped with ×40 objective (NA=1.25) on small pieces of the keel using natural lignin fluorescence for contrast to observe cell shape [29] and using fluorescence from safranine staining for contrast between the cell wall and CIL [27] . For safranine-stained samples, 10 μm of tissue was microtomed away from the top of cells to allow safranine to infiltrate the cell. For all samples, the laser excitation wavelength was 488 nm. Emissions were collected with the filter set to 530–600 nm for lignin autofluorescence and with two channels set to 515–545 nm and 590–700 nm for safranine stained samples. Enzyme treatments To investigate the role of the CIL in keel actuation, it was removed by enzymatic treatment as described previously [22] . Briefly, FCA-stained sections of keel (30 μm) were treated with Cellulase ONOZUKA RS from Trichoderma viride (EC 3.2.1.4) (2.3 enzyme units per mg) (Yakult Pharmaceutical Industry.) Samples were placed in Eppendorf tubes filled with a 1 ml of solution of 100 mg ml −1 enzyme in ammonium formate buffer (pH 5) and were placed in shaking water bath (40 °C, 60 r.p.m.) for 10 h. As a control, two samples were prepared and stained the same way but were treated only in 1 M ammonium formate (pH 5). The swelling behaviour of the cells was measured as described above. Finite element modelling A simplified finite element model of the keel-backing system was made using Abaqus 6.9 ( http://www.simulia.com ). Dimensions were chosen to be similar to the measured dimensions ( Fig. 4e ). Uniform isotropic linear elasticity was assumed with the same elastic coefficients for both the keel and the backing. The elastic coefficients were assumed to remain constant during swelling. The model was discretized using 7,900 hexahedral 8-node linear stress-displacement elements (C3D8). Mesh-size independence of the results was confirmed by running simulations with finer mesh (33,445 elements). A contractile longitudinal eigenstrain of 50% was simulated in the keel by applying a temperature change of 1 to 0 assuming only the keel has a thermal expansion coefficient of 0.5 in the longitudinal direction. No contraction was assumed in the transverse direction. As the elastic coefficients were chosen to be the same for both the keel and backing, the calculated deformation should be independent of the modulus. This was confirmed by performing simulations with elastic moduli ranging from 0.1 to 10 GPa with a Poisson's ratio of 0.3. How to cite this article: Harrington, M. J. et al . Origami-like unfolding of hydro-actuated ice plant seed capsules. Nat. Commun. 2:337 doi: 10.1038/ncomms1336 (2011).